Self-catalysed aerobic oxidization of organic linker in porous crystal for on-demand regulation of sorption behaviours Control over the structure and property of synthetic materials is crucial for practical applications. Here we report a facile, green and controllable solid–gas reaction strategy for on-demand modification of porous coordination polymer. Copper(I) and a methylene-bridged bis-triazolate ligand are combined to construct a porous crystal consisting of both enzyme-like O 2 -activation site and oxidizable organic substrate. Thermogravimetry, single-crystal X-ray diffraction, electron paramagnetic resonance and infrared spectroscopy showed that the methylene groups can be oxidized by O 2 /air even at room temperature via formation of the highly active Cu(II)-O 2 ˙− intermediate, to form carbonyl groups with enhance rigidity and polarity, without destroying the copper(I) triazolate framework. Since the oxidation degree or reaction progress can be easily monitored by the change of sample weight, gas sorption property of the crystal can be continuously and drastically (up to 4 orders of magnitude) tuned to give very high and even invertible selectivity for CO 2 , CH 4 and C 2 H 6 . Compared with conventional adsorbents, porous coordination polymers (PCPs) are unique for their diversified and tailorable coordination frameworks [1] , [2] , [3] , [4] , [5] , [6] , [7] , [8] , [9] , [10] , [11] . While tailoring structure/property generally refers to design/synthesis of new ligands and frameworks, some PCP prototypes can adopt several different metal ions and/or ligands, providing a rational strategy for adjusting the structure/property, albeit only in a limited degree [5] , [8] , [12] , [13] , [14] . A few of these prototypes can even form mixed-component (solid-solution) crystals with variable concentration/ratio of functional building blocks, which in principle allows the structure/property to be adjusted more continuously and precisely [15] , [16] . However, so far there is no rational strategy to directly monitor/control the composition of solid-solution frameworks during the synthesis process because complicated reaction environments involving solvents and/or liquid reactants are generally required for known direct-synthesis and post-synthetic modification (PSM) [3] , [7] , [17] , [18] , [19] , [20] , [21] methods. It should be noted that the reaction time/feeding ratio can be hardly used as a parameter for precise control over the reaction progress/framework composition, since the two variables have complicated relationships. Single-crystal X-ray diffraction is straightforward for direct visualization of the physical adsorption and chemical reaction events in PCPs [22] , but retaining the sample single crystallinity after physical/chemical changes is always a great challenge [22] , [23] , [24] , [25] , [26] , and crystallography is not a technique for quantitative analysis. If a PCP crystal could react with a gas (O 2 is a good yet difficult candidate) in the absence of assistant solvent/liquid, the sample weight or gas pressure can serve as an easily measurable parameter directly and linearly associated with its framework composition. The selective and ‘green’ oxidation of organic molecules by air or dioxygen (O 2 ) is fundamental in the biosystem and has long been pursued in industry and chemical sciences [27] , [28] , [29] . Because the energy barrier for electron transfer from singlet organic substrates to the triplet O 2 is generally very high [30] , harsh reaction conditions and/or efficient catalysts are usually necessary to activate the O 2 molecule for aerobic oxidization, so that the earth atmosphere can maintain a high O 2 concentration. Natural enzymes are well known as highly selective and efficient catalysts under mild conditions. For instance, the highly efficient O 2 activation centres in various copper proteins, such as galactose oxidase, tyrosinase and dopamine β -monooxygenase, have been extensively studied or used as structural models for synthetic catalysts. Considering that PCPs generally lack sufficient robustness, reactivity and/or O 2 -activation ability to allow aerobic oxidation of themselves, we designed and synthesized a porous metal azolate framework (MAF) [4] on the basis of Cu(I) and a methylene-bridged bis-triazolate ligand ( Fig. 1 ). Although Cu(I)-based PCPs are very scarce because Cu(I) can be easily oxidized as Cu(II) by air to destroy the original metal–ligand connectivity [31] , azolate derivatives have been demonstrated as suitable ligands for highly stable PCPs even with Cu(I) (ref. 4 ), and the coordination between Cu(I) and triazolate can be expected to give low-coordinated metal centres similar to those in the O 2 -activating copper proteins. Furthermore, the methylene bridge in a diarylmethane-type ligand is obviously flexible and oxidizable (activated by two aromatic rings) [32] , which could be oxidized in suitable catalytic conditions to form a more rigid and polar ketone group. 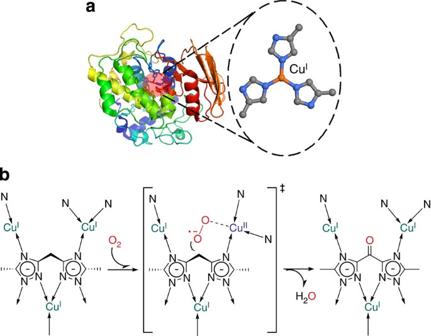Figure 1: Bioinspired aerobic oxidation strategy for multifunctional porous frameworks. (a) The O2-activating site in a typical copper protein. (b) The possible coordination structure and reactivity of an extended network solid (porous crystal) consisting of Cu(I) and a methylene-bridged bistriazolate ligand. Figure 1: Bioinspired aerobic oxidation strategy for multifunctional porous frameworks. ( a ) The O 2 -activating site in a typical copper protein. ( b ) The possible coordination structure and reactivity of an extended network solid (porous crystal) consisting of Cu(I) and a methylene-bridged bistriazolate ligand. Full size image Preparation and characterization of the porous crystal Colourless crystals of the titled compound, MAF-42, were synthesized in its large-pore ( lp ) form as [Cu 4 (btm) 2 ]·C 6 H 6 (denoted as C 6 H 6 @MAF-42- lp , H 2 btm=bis(5-methyl-1,2,4-triazolate-3-yl)methane) by solvothermal reaction of H 2 btm and [Cu(NH 3 ) 2 ]OH in a mixed aqueous ammonia/methanol/benzene solvent. Single-crystal X-ray diffraction analysis ( Supplementary Table 1 ) showed that MAF-42- lp is a three-dimensional (3D) porous coordination framework composed of five independent (two of them locate at twofold axes with occupancies of 1/2) Cu(I) ions and two independent, fully deprotonated btm 2− ligands in a 2:1 molar ratio. As expected, all btm 2− ligands are six-coordinated and the average coordination number of Cu(I) ions is three [4] . Nevertheless, each Cu(I) ion either adopts the linear, distorted T-shaped or tetrahedral coordination geometry ( Supplementary Fig. 1 ). The two independent ligands have different surrounding environments. 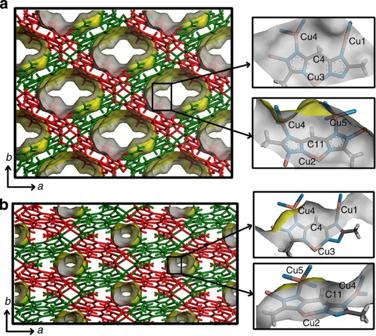Figure 2: Guest-induced framework breathing. (a) C6H6@MAF-42-lp(b) MAF-42-sp. The ribbon-like fragments of the coordination framework running along two directions are highlighted in green and red, respectively, and the pore surfaces of 1D channels are highlighted as yellow/grey curved planes. Desolvation leads to –28%, +10% and –22% changes ina,bandV, respectively. The methylene group (C4) of one ligand is adjacent to a two- and two three-coordinated Cu(I) ions, while that (C11) of another ligand is only adjacent to two three- and a four-coordinated Cu(I) ions ( Supplementary Table 2 ). The two triazolate rings of btm 2− are not coplanar because they are linked by a sp 3 hybridized methylene C atom. The 3D coordination framework can be regarded as a cross-packing structure of ribbon-like fragments ( Supplementary Fig. 2 ), which retains large 1D rhombic channels (void 37.8%, cross-section size 4.8 × 7.1–6.0 × 10.8 Å 2 ) with disordered benzene molecules filled inside. It should be noted that the Cu(I) ions and methylene groups are fully exposed on the pore surface ( Fig. 2a ). Figure 2: Guest-induced framework breathing. ( a ) C 6 H 6 @MAF-42- lp ( b ) MAF-42- sp . The ribbon-like fragments of the coordination framework running along two directions are highlighted in green and red, respectively, and the pore surfaces of 1D channels are highlighted as yellow/grey curved planes. Desolvation leads to –28%, +10% and –22% changes in a , b and V , respectively. Full size image Thermogravimetry (TG) and powder X-ray diffraction (PXRD) measurements of C 6 H 6 @MAF-42- lp showed that the benzene molecules can be completely removed below 260 °C to form the small-pore ( sp ) phase [Cu 4 (btm) 2 ] (denoted as MAF-42- sp or simplified as MAF-42), which can be stable up to 410 °C ( Supplementary Figs 3 and 4 ). Single-crystal structure of MAF-42- sp ( Supplementary Table 1 ) showed significantly contracted unit cell (–22%) and channel size (void 14.1%, cross-section size 2.4 × 2.6–3.5 × 3.7 Å 2 ) because the cross angle of packed ribbons reduced from 72° to 53° ( Fig. 2b ) [5] , [8] . In MAF-42- sp , the Cu(I) ions and methylene groups are less exposed on the pore surface; however, their separations are similar to those in MAF-42- lp ( Supplementary Table 2 ). While the coordination bond lengths were changed very little (Δ max =0.022 Å), the structural variation mainly occurred on the ligand conformations and coordination geometries of the Cu(I) ions serving as the joints between the ribbon-like fragments (Δ max =7.3°; Supplementary Tables 2 and 3 ). Actually, the ligand-bending directions are reversed, that is, the average torsion angle between two triazolate rings of btm 2− changes from 167.6° in MAF-42- lp to −165.1° in MAF-42- sp ( Supplementary Fig. 5 ). The structure transformation between C 6 H 6 @MAF-42- lp and MAF-42- sp can be reversibly triggered by adsorption/desorption of benzene vapour ( Supplementary Fig. 4 ). Self-catalysed aerobic oxidation In air, colourless C 6 H 6 @MAF-42- lp turns brown and then black quickly ( Fig. 3a ), which should not be originated from Cu(I) to Cu(II) oxidation because the Cu(II) complex is usually blue or green. Electrospray ionization mass spectrometry of the demetalated samples showed that fresh C 6 H 6 @MAF-42- lp has only a signal at m / z =179 (H 3 btm + ), while a new peak at m / z =193 corresponding to the expected oxidation product bis(5-methyl-1,2,4-triazol-3-yl)methanone (H 3 btk + ) appeared after the sample was exposed in air ( Supplementary Fig. 6 ). The infrared spectrum of the oxidized sample exhibits a strong band at 1641, cm −1 in the characteristic region of 1,750±150 cm −1 for carbonyl groups ( Supplementary Fig. 7 ). The single-crystal structure of a black crystal obtained by prolonged exposure (1 month) of C 6 H 6 @MAF-42- lp in air was measured ( Supplementary Table 1 ). A residual electron peak appeared near one of the two crystallographically independent methylene groups that adjacent to the two-coordinated Cu(I) ion, which can be refined as an oxygen atom without any restriction, giving an occupancy of 0.28(5) and a C=O bond length of 1.20(5) Å ( Supplementary Fig. 8 ) [33] . These observations demonstrated that the btm 2− ligands in C 6 H 6 @MAF-42- lp can be readily oxidized by air at room temperature, although the reaction rate is quite slow. The oxidation of MAF-42- sp (almost no colour change after exposed in air at room temperature for several days) is much slower, which may be ascribed to the even smaller pore size and less exposed active sites. 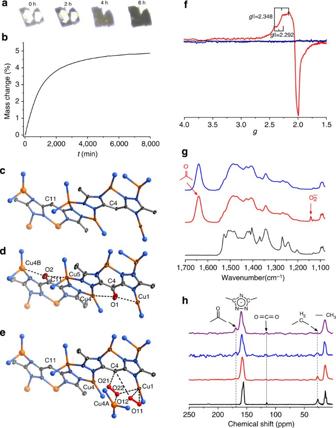Figure 3: Controlling the reaction degree and revealing the catalytic mechanism of aerobic oxidation. (a) Photographs of C6H6@MAF-42-lpexposed in air at room temperature for different time. (b) TG of MAF-42 in an O2flow at 418 K. (c–e) X-ray single-crystal structures of MAF-42,O65and O2@MAF-42 (probability drawn at 30% for independent atoms; symmetric codes: A=1−x, −y, 1−z; B=x, 1−y, −0.5+z). The black dashed lines are drawn to highlight relatively short nonbonding interactions (Cu1···O11 3.04(4) Å, Cu1···O12 3.28(3) Å, Cu4···O22 3.73(6) Å), C4···O12 4.47(6) Å, C4···O21 3.46(6) Å, Cu1···O1 2.61(1) Å, Cu4···O2 2.79(1) Å). (f) EPR spectra of MAF-42 in O2measured at 298 K (black) and then at 473 K (red) and then back to 298 K (blue). (g) DR-FTIR spectra of MAF-42 measured at 473 K under a variable atmosphere from helium (black) to oxygen (red) and then back to helium (blue). (h) Solid-state13C NMR spectra of MAF-42 (black),O53(red),O74(blue) andO100(purple). Figure 3: Controlling the reaction degree and revealing the catalytic mechanism of aerobic oxidation. ( a ) Photographs of C 6 H 6 @MAF-42- lp exposed in air at room temperature for different time. ( b ) TG of MAF-42 in an O 2 flow at 418 K. ( c – e ) X-ray single-crystal structures of MAF-42, O65 and O 2 @MAF-42 (probability drawn at 30% for independent atoms; symmetric codes: A=1− x , − y , 1− z ; B= x , 1− y , −0.5+ z ). The black dashed lines are drawn to highlight relatively short nonbonding interactions (Cu1···O11 3.04(4) Å, Cu1···O12 3.28(3) Å, Cu4···O22 3.73(6) Å), C4···O12 4.47(6) Å, C4···O21 3.46(6) Å, Cu1···O1 2.61(1) Å, Cu4···O2 2.79(1) Å). ( f ) EPR spectra of MAF-42 in O 2 measured at 298 K (black) and then at 473 K (red) and then back to 298 K (blue). ( g ) DR-FTIR spectra of MAF-42 measured at 473 K under a variable atmosphere from helium (black) to oxygen (red) and then back to helium (blue). ( h ) Solid-state 13 C NMR spectra of MAF-42 (black), O53 (red), O74 (blue) and O100 (purple). Full size image The TG analysis showed that heating microcrystalline MAF-42- sp in an O 2 flow at 418 K could be an optimized reaction condition, in which complete oxidation can be achieved after ~8,000 min ( Fig. 3b ). Meanwhile, mass spectrometry analysis of the effluent showed that water is produced as a byproduct during the oxidation process ( Supplementary Fig. 9 ). Therefore, on the basis of the simple reaction equation ( Fig. 1b ), the oxidation degree of the crystals can be simply calculated and controlled by the heating time or by monitoring the sample weight. The PXRD pattern of the fully oxidized sample is similar to that of MAF-42- sp ( Supplementary Fig. 10 ), indicating the retention of the original framework connectivity. X-ray photoelectron spectroscopy showed that, even on the particle surface of the oxidized sample, only very small amounts of Cu(I) ions have been oxidized to Cu(II) ( Supplementary Fig. 11 ). While some oxidation reactions have been used to modify the organic linkers in PCP crystals, strong and environment-unfriendly oxidants (such as nitric acid and dimethyldioxirane), as well as organic solvents are necessary [17] , [18] , [34] , [35] , [36] . Compared with the conventional oxidation methods, the solvent-free aerobic oxidation is obviously much greener yet more difficult. At the same conditions, the free ligand H 2 btm cannot be oxidized ( Supplementary Fig. 12 ), highlighting the difficulty of covalent redox PSM and crucial role of enzyme-like Cu(I) centres. Compared with known direct-synthesis and PSM methods, the aerobic oxidation is also noteworthy for its controllable, solvent-free and solid–gas reaction mechanism, which can be conveniently used to tailor the adsorbent properties. Interestingly, the oxidized samples can be completely reduced back to C 6 H 6 @MAF-42- lp by hydrazine ( Supplementary Fig. 13 ). The structure of a highly oxidized single crystal [Cu 4 (btm) 0.7 (btk) 1.3 ] (denoted as O65 to reflect the oxidation degree, 65%) has been successfully measured ( Supplementary Table 1 ). There are residual electron peaks near the two independent methylene groups, which were refined as oxygen atoms to give occupancies of 0.73(2) and 0.57(2) and C=O bond lengths of 1.236(10) and 1.234(11) Å, respectively ( Fig. 3c,d ). Again, the oxidation degree of methylene near the two-coordinated Cu(I) is higher. In O65 , weak Cu(I)-carbonyl interactions can be observed ( Supplementary Table 2 ), which are consistent with the relatively low wave number of carbonyl absorption in the infrared spectrum. Such unambiguous crystallography evidence is noteworthy because the harsh reaction condition for covalent PSM generally degrades crystallinity so that the modification degree is not high enough to be determined by crystal-structure analysis [23] , [37] , [38] . O65 has a slightly smaller and distorted unit cell compared with MAF-42- sp (Δ V / V 1 =−0.6%, Δ β =−1.0°), which can be ascribed to the generation of polar carbonyl groups on the pore surface and dipole–dipole attractive interactions within the host framework of O65 . While the unit-cell volume follows C 6 H 6 @MAF-42- lp >> MAF-42- sp > O65 , their organic ligands deviate from the planar conformation by 12.4, −14.9 and −12.9°, respectively ( Supplementary Fig. 5 ). Obviously, oxidation enhances the conjugation degree and planarity of ligands, which are disadvantageous for framework contraction. To further shrink from MAF-42- sp to O65 , the coordination bonding lengths (Δ max =0.044 Å) and angles (Δ max =9.6°) are forced to change more ( Supplementary Tables 2 and 3 ). On the other hand, framework contraction also reduces the planarity of ligands in O65 . To gain more insight into the aerobic oxidation process, we tried to capture some reaction intermediates. In the single-crystal structure of MAF-42 loaded with O 2 (denoted as O 2 @MAF-42) at low temperature of −140 °C ( Supplementary Table 1 ), although O 2 molecules are highly disordered, it can be seen that the primary adsorption sites are close to the two- and three-coordinated Cu(I) ions and the methylene group having a preference for oxidation ( Fig. 3e and Supplementary Table 2 ). The presence of Cu(II) species during the aerobic oxidation reaction was confirmed by the axially symmetric signal with g || =2.292~2.348 and the vertical signal with g ⊥ =2.089 in the in situ electron paramagnetic resonance (EPR) spectroscopy measured at 200 °C ( Fig. 3f ) [39] . Because the peak intensity at g ~2.0–2.3 originated from the Cu(II) ion is vastly greater than that of the radical O 2 ˙− at g ~2, the latter is difficult to assign. On the other hand, in situ diffuse reflectance-Fourier transform infrared spectroscopy showed absorption bands at 1,140 cm −1 characteristic for the O 2 ˙− species ( Fig. 3g ) and 458 cm −1 characteristic for the Cu–O coordination bond ( Supplementary Fig. 14 ) [40] . The observation of physical adsorption at low temperature and chemical adsorption at high temperature is similar with some other heterogeneous reactions involving gas reactants and solid catalysts [41] . Therefore, some key stages of the aerobic oxidation mechanism have been observed, in which O 2 molecules first attack the low-coordinated Cu(I) ions, and then form the highly active intermediate Cu(II)-O 2 ˙− reactive enough to break the hydrocarbon C–H bond, and finally returned to Cu(I) and produced the carbonyl product and water. The reaction can be unambiguously assigned to the Cu(II)/Cu(I) redox couple and metal-centred four-electron oxidation mechanism, which are commonly expected for natural enzymes and small molecular complexes but have been scarcely confirmed [18] , [19] . The catalytic activity of the low-coordinated Cu(I) sites in MAF-42 for aerobic oxidation of guest reactants was further confirmed by its effectiveness and low activation energy for the reaction of CO+O 2 =CO 2 ( Supplementary Methods , Supplementary Figs 4 and 15 ). Regulation of gas adsorption properties To reveal the structure–property relationship, MAF-42 was oxidized to different degrees by the above established aerobic oxidation method. By virtue of the solid–gas reaction mechanism, the products were obtained in quantitative yields and were used without further workup procedure. Solid-state 13 C nuclear magnetic resonance (NMR) spectra showed that the methylene peak at 27 p.p.m. and carbonyl peak at 169 p.p.m. gradually reduces and increases, respectively, as the oxidation degree increases ( Fig. 3h ). On the basis of the peak areas of the methylene (2.8 p.p.m.) and methyl (0.8 p.p.m.) groups observed in the solution 1 H NMR spectra of the DCl-digested samples ( Supplementary Fig. 16 ), the oxidation degrees of the oxidized samples (hereafter denoted as O53 , O74 and O100 , respectively) were calculated as 53%, 74% and 100%. PXRD and TG showed that oxidization enhances the hydrophilicity, decreases the thermal stability and reduces the unit-cell volumes of the samples ( Supplementary Figs 17 and 18 ), being consistent with the generation of more polar carbonyl groups [4] . Single-component CO 2 isotherms were measured for MAF-42, O53 , O74 and O100 at 195 K to characterize their porosity and framework flexibility/rigidity, which all exhibited hysteresis ( Fig. 4a and Supplementary Fig. 19a ). The isotherm of MAF-42 showed a direct transition from the nonporous ( np ) phase ( P / P 0 <0.25) to the lp phase ( P / P 0 >0.40). The absence of the sp phase in the isotherm of MAF-42 can be explained by its extremely small aperture size (2.2 × 2.6 Å 2 ) and inert pore surface. 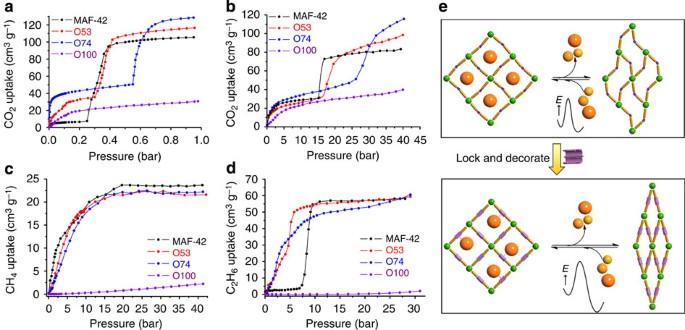Figure 4: Modulation of single-component gas adsorption properties. (a) CO2at 195 K. (b) CO2at 298 K. (c) CH4at 298 K. (d) C2H6at 298 K. Lines are drawn to guide eyes. (e) Elucidation of the gas adsorption mechanism. The framework flexibility and pore surface polarity of a porous crystal are modulated by chemical modification of the organic linker. Specifically, for MAF-42, the hydrophobic and flexible methylene bridges are transformed to hydrophilic and rigid carbonyl ones via aerobic oxidation, and the transformation ratio is controlled by the oxidation degree. Differently, O53 and O74 exhibited the expected sp -to- lp transition, as their first-step saturation uptakes are coincident with the theoretical values calculated from the crystal structures of MAF-42 and O65 ( Supplementary Table 4 ). The increased CO 2 -binding ability of the oxidized samples is consistent with their enhanced pore surface polarity. The second-step saturation uptake and the corresponding pore volume follow O74 (128 and 0.23 cm 3 g −1 ) > O53 (116 and 0.21 cm 3 g −1 ) >MAF-42 (105 and 0.19 cm 3 g −1 ), indicating that oxidization can expand the lp phase of the host frameworks, which was further quantified by the unit-cell volumes of guest-saturated samples ( Supplementary Fig. 20 ). Framework expansion of the lp phase could be ascribed to the enhanced rigidity of the oxidized ligand, which usually increases the bridging length. In the lp phase, the dipole–dipole attraction effect (causing the shrinkage of the sp phase [42] ) can be eliminated by insertion of guest in the channels [5] , [8] . Figure 4: Modulation of single-component gas adsorption properties. ( a ) CO 2 at 195 K. ( b ) CO 2 at 298 K. ( c ) CH 4 at 298 K. ( d ) C 2 H 6 at 298 K. Lines are drawn to guide eyes. ( e ) Elucidation of the gas adsorption mechanism. The framework flexibility and pore surface polarity of a porous crystal are modulated by chemical modification of the organic linker. Specifically, for MAF-42, the hydrophobic and flexible methylene bridges are transformed to hydrophilic and rigid carbonyl ones via aerobic oxidation, and the transformation ratio is controlled by the oxidation degree. Full size image More interestingly, when the oxidation degree increases, the gate-opening/closing pressure (defined as the intermediate pressure between two isotherm steps) increases during adsorption ( P / P 0 =0.32, 0.35 and 0.74 for MAF-42, O53 and O74 , respectively) but decreases during desorption ( P / P 0 =0.25, 0.21 and 0.14 for MAF-42, O53 and O74 , respectively) to widen the hysteresis loop, which demonstrates that oxidization increases the ligand rigidity and difficulty of phase transition and the oxidized samples are solid-solution frameworks rather than mechanical mixtures [15] , [43] . Further, O100 showed one-step sorption isotherm with a small saturation uptake of ca 30 cm 3 g −1 ( Fig. 4a and Supplementary Fig. 19a ), confirming that it’s sp phase has the most shrunk structure compared with the counterparts with lower oxidation ratios, and is too rigid to undergo the sp -to- lp transition. Therefore, the oxidized framework exhibited larger breathing amplitude, energy change and energy barrier during sp -to- lp transition. Only a couple of examples have demonstrated the control of framework flexibility by PSM of PCPs [42] , [44] , in which different functional building blocks were added into the coordination framework, which always reduced the pore volume and the regulation is uncontrollable and discontinuous. In our case, the aerobic oxidation has negligible size effect (similar for methylene and carbonyl) but directly increases the ligand/framework rigidity and the pore volume of the lp phase, so that the oxidized framework exhibits enhanced adsorption capacity. More importantly, the solid–gas reaction mechanism allows modification ratio and gas sorption property to be continuously and conveniently monitored/controlled. High-pressure single-component CO 2 , C 2 H 6 and CH 4 sorption isotherms were measured at 298 K ( Fig. 4b–d and Supplementary Fig. 19b–d ). The room-temperature CO 2 sorption isotherms are similar to those measured at 195 K, except that MAF-42 shows the sp -to- lp transition at room temperature. The abnormal temperature-dependent sorption behaviour of the sp phase of MAF-42 can be ascribed to thermal expansion ( Supplementary Fig. 4 ) and/or decreased diffusion barrier [45] . The gradually increased gate-opening pressure (16, 18, 28 and >40 bar for MAF-42, O53 , O74 and O100 , respectively) and decreased isotherm slope of the sp -to- lp transition are consistent with the increased framework rigidity of the oxidized samples ( Fig. 4e ). For CH 4 , MAF-42, O53 and O74 show type-I adsorption isotherms corresponding to the sp phase ( Supplementary Table 4 ). 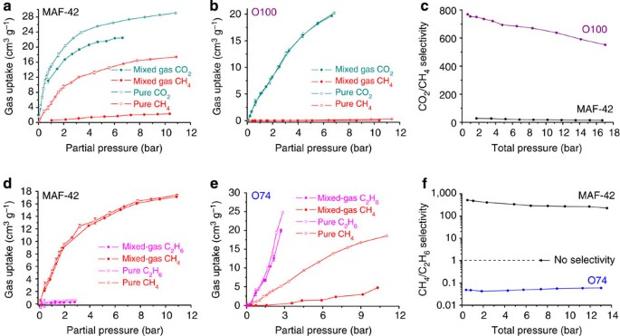Figure 5: Modulation of mixed-gas adsorption selectivity. (a–c) A ratio of 40:60 CO2/CH4for MAF-42 andO100, as well as the corresponding CO2/CH4selectivity. (d–f) A ratio of 80:20 CH4/C2H6for MAF-42 andO74, as well as the corresponding CH4/C2H6selectivity. All gas adsorption isotherms were measured at 298 K. Lines are drawn to guide eyes. Compared with CO 2 , CH 4 has very low boiling point and polarity ( Supplementary Table 5 ), meaning that it interacts with the host framework very weakly and can hardly open the narrow channel or induce the sp -to- lp transition. The variation of C 2 H 6 sorption isotherms of MAF-42, O53 and O74 resembles that of CO 2 at 195 K. The gate-opening pressure is 8 bar for the np -to- lp transition of MAF-42, which is higher than those of 5 and 6 bar for the sp -to- np transitions of O53 and O74 , respectively. The nonporous sp phase of MAF-42 for C 2 H 6 can be explained by the very large molecular size of the guest ( Supplementary Table 5 ). Because of the over-shrinkage of the host framework, O100 is virtually nonporous for the low-polarity gases CH 4 and C 2 H 6 . The finely/drastically tunable gas sorption properties suggest their usefulness for on-demand gas separation. Mixed gas adsorption isotherms were measured to reveal the real gas adsorption selectivities of selected samples with promising isotherms. The CO 2 /CH 4 selectivities of MAF-42 and O100 at 1–10 bar (measured by mixed CO 2 /CH 4 with 40:60 molar ratio) were observed as 28–14 and 700–600, respectively ( Supplementary Methods , Fig. 5a–c ), meaning that the performance of the crystal can be significantly improved by the aerobic oxidation treatment. The extremely high CO 2 /CH 4 selectivity of O100 should be suitable for purifying CH 4 from biogases (CH 4 45~65%, CO 2 30~50%) [46] and landfill gases (CH 4 35~55%, CO 2 40~45%) [47] by selective adsorption of CO 2 . Figure 5: Modulation of mixed-gas adsorption selectivity. ( a – c ) A ratio of 40:60 CO 2 /CH 4 for MAF-42 and O100 , as well as the corresponding CO 2 /CH 4 selectivity. ( d – f ) A ratio of 80:20 CH 4 /C 2 H 6 for MAF-42 and O74 , as well as the corresponding CH 4 /C 2 H 6 selectivity. All gas adsorption isotherms were measured at 298 K. Lines are drawn to guide eyes. Full size image More interestingly, the real CH 4 /C 2 H 6 selectivities (measured by mixed CH 4 /C 2 H 6 with 20:80 molar ratio) were observed to be 500–200 and 1/24–1/17 for MAF-42 and O74 , respectively, indicating the catalytic oxidation can drastically invert the CH 4 /C 2 H 6 selectivity up to 4 orders of magnitude, which has not been realized by other adsorbents or methods ( Supplementary Methods , Fig. 5d–f ). The selective adsorption of CH 4 by MAF-42 at low pressure is due to its nonporous nature for C 2 H 6 according to the molecular sieving effect. On the other hand, O74 prefers adsorption of C 2 H 6 because it is porous to both gases, and C 2 H 6 has the larger molecular weight and quadrupole moment ( Supplementary Table 5 ). This property may be useful for on-demand purification of different mixture gases (for example, natural gases usually contain CH 4 69~96% and C 2 H 6 1~14%) [2] , [48] . Conventional adsorbents generally exhibit Langmuir-type isotherm and monotonically decreased (versus pressure) adsorption selectivity, which is not suitable for some gas separation applications operating at high pressures [49] . Some flexible PCPs showing gate-opening phenomena and stepped isotherms may be used to solve this problem; however, the real selectivities are usually much lower than those predicted by the single-component isotherms because the non-preferred guest can also enter the opened channel above the gate-opening pressure [50] . We observed that the real C 2 H 6 /CH 4 selectivity (measured by mixed C 2 H 6 /CH 4 with 75:25 molar ratio) of O53 significantly increases from 92 to 140 at C 2 H 6 partial pressure from 4.7 to 5.5 bar, respectively, and remains 113 at C 2 H 6 partial pressure of 8.1 bar ( Supplementary Methods and Supplementary Fig. 21 ). The abrupt increase in real adsorption selectivity occurs around the gate-opening pressure of single-component C 2 H 6 isotherm at 4.7–5.2 bar. This observation indicates that the gate-opening is forced by filling the C 2 H 6 molecules in the newly generated space. In other words, there is no space left for CH 4 , preventing the commonly observed co-adsorption effect. In summary, we demonstrated that Cu(I) ions with enzyme-like O 2 activation ability can cooperate with a flexible and oxidizable bis-triazolate ligand to fabricate a porous crystal reactive towards molecular oxygen even at room temperature. The methylene bridge of the bis-triazolate ligand provides the key reactivity to molecular oxygen, as well as modifiable framework flexibility and pore surface polarity. Although the free ligand is inert to oxygen, the flexible methylene bridge near the low-coordinated Cu(I) centres in the coordination framework is reactive enough to be oxidized as a more rigid and polar carbonyl group. In situ structural and spectroscopic analyses confirmed that the low-coordinated Cu(I) centres behave like those in copperproteins during the aerobic oxidation. Compared with known material synthesis and processing methods, the solvent-free aerobic oxidation reaction has a series of advantages, such as green, quantitative yield, easy and precise monitor/control of modification degree, work-up procedure free, and so on. While conventional adsorbents separate adsorbates with fixed selectivities by either sorption affinity difference or molecular sieving effect, the porous crystal consisting of a reactive organic linker with modifiable flexibility and polarity offers a possibility to utilize both mechanisms, as demonstrated by the very high, drastically tunable and even switchable gas sorption selectivities. These results may enlighten future design and construction of multifunctional and controllable porous materials. Materials Commercially available reagents and solvents were used without further purification. The ligand H 2 btm was synthesized according to the literature method [51] . Measurements Infrared spectra were obtained from KBr pellets on a Bruker TENSOR 27 FT IR spectrometer in the 400- to 4,000-cm –1 region. Diffused reflection Fourier transform infrared spectroscopy (DR-FTIR) was performed on a Bruker VERTEX 70 spectrometer in the 400- to 4,000-cm –1 region. TG-mass spectra were performed on a hyphenated apparatus of NETZSCH STA 449 F3 Jupiter and NETZSCH QMS 403C Aedo. Elemental analyses (C, H and N) were performed with a Vario EL elemental analyser. TG analyses were performed by using a TA Q50 system. Solid-state 13 C NMR measurements were carried out at ambient temperature on a Bruker AVANCE 400 spectrometer. Solution 1 H NMR measurements were carried out at ambient temperature on a VARIAN Mercury-Plus 300 spectrometer, for which ~20 mg of solid samples were digested with sonication in 550 μl of DCl (20 wt% in D 2 O). PXRD patterns were collected (0.02° per step, 0.06 s per step except for otherwise stated) on a Bruker D8 Advance diffractometer (Cu Kα) at room temperature. Mass spectra were measured by a SHIMADZU LCMS-2010A equipment using an electrospray ionization source with MeOH as the mobile phase. Electron paramagnetic resonance measurements were performed at 9.7 GHz (X-band) using a Bruker BioSpin A300 spectrometer. The spin concentrations in the samples were determined from the second integral of the spectra using CuSO 4 ·5H 2 O as a standard. The as-synthesized sample (weight of ~100−200 mg) was placed in the self-made quartz tube and dried for 8 h at 260 °C under high vacuum to remove the remnant solvent molecules, sealed with back-filled O 2 before measurements. Synthesis of materials A mixture of aqueous ammonia (25%, 4 ml) solution of [Cu(NH 3 ) 2 ]OH (0.025 mol l −1 ), H 2 btm (0.009 g, 0.05 mmol), methanol (3.0 ml) and benzene (1.0 ml) was sealed in a 15-ml Teflon-lined stainless reactor, which was heated in an oven at 160 °C for 72 h. The oven was cooled to room temperature at a rate of 5 °C h −1 . The resulting colourless block crystals were filtered, washed by ethanol and dried in air to give C 6 H 6 @MAF-42- lp (yield ca 83%). Guest-free MAF-42 was obtained by heating C 6 H 6 @MAF-42- lp at 260 °C under high vacuum for 24 h. The oxidized samples were obtained by heating MAF-42 at 418 K in the O 2 flow for different times. X-ray crystallography Single-crystal diffraction intensities were collected on a Bruker Apex CCD diffractometer with graphite-monochromated Mo Kα radiation or a Oxford Gemini S Ultra CCD diffractometer using mirror-monochromated Cu Kα radiation. Absorption corrections were applied by using the multiscan programme SADABS. The structures were solved by the direct method and refined with a full-matrix least-squares technique with the SHELXTL 6.10 programme package. The occupancies of carbonyl oxygen atoms and guest molecules were obtained by free refinement. Anisotropic thermal parameters were applied to all non-hydrogen atoms of host frameworks except for the oxygen atom in structure obtained by prolong exposure of C 6 H 6 @MAF-42- lp in air. Hydrogen atoms were generated geometrically. Crystal data for the complexes were summarized in Supplementary Table 1 . PXRD data for Pawley refinement were collected in 0.02° per step and 3 s per step. Indexing and Pawley refinement of the PXRD patterns was carried out by using the Reflex module of Material Studio 5.0. The patterns were indexed by the TREOR90 method with the aid of unit-cell parameters from single-crystal data. Pawley refinements were carried out with the cell parameters obtained from indexing in space group C 2/ c . Peak profiles, zero-shifts and unit-cell parameters were refined simultaneously. The peak profiles were refined by the Pseudo-Voigt function with Berar–Baldinozzi asymmetry correction parameters. Gas sorption measurement and calculation The single-component gas sorption isotherms were measured with automatic volumetric adsorption apparatuses (BELSORP-max and BELSORP-HP). The mixed gas adsorption isotherms were measured by volumetric adsorption−gas chromatograph instrument BELSORP-VC with a maximum measurement pressure of 15 bar. The as-synthesized sample (weight of ~500−800 mg) was placed in the quartz tube and dried for 8 h at 260 °C to remove the remnant solvent molecules before measurements. CO 2 (99.999%), CH 4 (99.999%) and C 2 H 6 (99.99%) were used for all measurements. The temperatures were controlled by an acetone−dry ice bath (195 K) or a water bath (298 K). Accession codes. The X-ray crystallographic coordinates for structures reported in this Article have been deposited at the Cambridge Crystallographic Data Centre (CCDC), under deposition number CCDC 1041776–1041780. These data can be obtained free of charge from The Cambridge Crystallographic Data Centre via www.ccdc.cam.ac.uk/data_request/cif . How to cite this article: Liao, P.-Q. et al. Self-catalysed aerobic oxidization of organic linker in porous crystal for on-demand regulation of sorption behaviours. Nat. Commun. 6:6350 doi: 10.1038/ncomms7350 (2015).